HOP2-MND1 modulates RAD51 binding to nucleotides and DNA The HOP2-MND1 heterodimer is required for progression of homologous recombination in eukaryotes. In vitro , HOP2-MND1 stimulates the DNA strand exchange activities of RAD51 and DMC1. We demonstrate that HOP2-MND1 induces changes in the conformation of RAD51 that profoundly alter the basic properties of RAD51. HOP2-MND1 enhances the interaction of RAD51 with nucleotide cofactors and modifies its DNA-binding specificity in a manner that stimulates DNA strand exchange. It enables RAD51 DNA strand exchange in the absence of divalent metal ions required for ATP binding and offsets the effect of the K133A mutation that disrupts ATP binding. During nucleoprotein formation HOP2-MND1 helps to load RAD51 on ssDNA restricting its dsDNA-binding and during the homology search it promotes dsDNA binding removing the inhibitory effect of ssDNA. The magnitude of the changes induced in RAD51 defines HOP2-MND1 as a ‘molecular trigger’ of RAD51 DNA strand exchange. The homologous recombination (HR) pathway plays an important role in the maintenance of genome integrity. The HR machinery is responsible for the repair of DNA double-strand breaks (DSBs), the restart of stalled replication forks, maintenance of telomeres and the accurate segregation of homologous chromosomes during meiosis [1] , [2] , [3] , [4] , [5] , [6] , [7] , [8] , [9] . Generally, HR is initiated by the formation of DSBs induced by various agents including ionizing radiation, reactive chemicals and the meiosis-specific protein Spo11 (ref. 10 ). DSBs are first processed exonucleolytically to generate 3′ ssDNA tails. Then, DNA recombinases of the RecA protein family bind this tailed DNA forming nucleoprotein filaments that perform the search for homologous dsDNA and DNA strand exchange. We and others showed that bacterial RecA, the best studied member of the recombinase family, has two DNA-binding sites, the primary and secondary, located in the region of L1 and L2 disordered loops [11] , [12] , [13] , [14] . The initial binding of ssDNA during nucleoprotein filament formation occurs in the primary site, while the secondary site is involved in interaction with dsDNA during the search for homology [15] , [16] , [17] . In most eukaryotes including humans, DNA strand exchange is promoted by RAD51 and DMC1 recombinases, structural and functional homologues of the bacterial RecA protein [18] . RAD51 is important for both mitotic and meiotic recombination, whereas DMC1 functions only during meiosis [19] , [20] , [21] , [22] , [23] . The HR pathway also includes auxiliary proteins that assist RAD51 and DMC1 in various recombination events [7] , [24] . It was shown that the Hop2 and Mnd1 proteins, which form a stable heterodimer, are required for normal progression of meiotic recombination [25] , [26] , [27] , [28] , [29] , [30] . In both yeast and mice, inactivation of HOP2-MND1 results in meiotic arrest, deficiency in the repair of meiotic DSBs and in aberrant synapsis between non-homologous chromosomes. In Hop2 knockout mice, RAD51/DMC1 form nuclear foci, indicating normal initiation of HR; however, these foci persist much longer than in wild-type cells, consistent with the inability of RAD51/DMC1 to promote DNA strand invasion in the absence of HOP2-MND1 (ref. 25 ). In higher eukaryotes, HOP2 and MND1 besides their meiotic function likely posses a DNA repair function during vegetative cell growth since both proteins are expressed in somatic tissues in plants, mice and humans [27] , [31] , [32] . In vitro , it was shown that HOP2-MND1 stimulates the DNA strand exchange activity of DMC1 and RAD51 (refs 28 , 33 , 34 , 35 , 36 , 37 , 38 ). Given the critical role of HR in accurate chromosome segregation and maintenance of genome stability, the mechanism of this stimulation is of significant interest. Biochemical analysis demonstrated that HOP2-MND1 stabilizes the RAD51- and DMC1-ssDNA nucleoprotein filament and stimulates the capture of dsDNA by the nucleoprotein filament, two pre-requisites for efficient recombinase-mediated homology search and strand exchange [36] , [37] , [38] . However, the underlying molecular basis for these effects of HOP2-MND1 on RAD51/DMC1 remains to be investigated. Our current data demonstrate that in mammals HOP2-MND1 induces changes in the RAD51 conformation, which have a profound effect on properties of RAD51 activating it for DNA strand exchange. HOP2-MND1 helps to preserve the RAD51-ssDNA filament in an active form countering the accumulation of ADP generated during ATP hydrolysis by RAD51. HOP2-MND1 enhances the interaction of RAD51 with nucleotide cofactors enabling RAD51 DNA strand exchange in the absence of divalent metal ions that are normally required for ATP binding. Also, the current results show that HOP2-MND1 strongly affects the specificity of DNA binding by increasing the RAD51 binding preference for ssDNA compared with dsDNA during the formation of the nucleoprotein filament. Furthermore, HOP2-MND1 modulates the interaction of the RAD51-ssDNA filament with DNA during the search for homology rendering DNA strand exchange insensitive to inhibition by ssDNA. Thus, HOP2-MND1 shows an unprecedented ability to stimulate DNA strand exchange by modulating a range of RAD51 basic properties, particularly nucleotide and DNA binding. HOP2-MND1 does not affect RAD51-ADP accumulation It was previously found that ATP hydrolysis by a human RAD51 (hRAD51) nucleoprotein filament in the presence of Mg 2+ leads to the rapid accumulation of hRAD51–ADP–ssDNA complexes concomitant with the loss of DNA strand exchange activity [39] . On the other hand, Ca 2+ by inhibiting the hRAD51 ATPase preserves the filament in an ATP-bound form that is active in DNA strand exchange [39] . Here we investigated whether HOP2-MND1 that stimulates the hRAD51 DNA strand exchange activity in the presence of Mg 2+ can also suppress accumulation of hRAD51–ADP–ssDNA complexes. To test the effect of HOP2-MND1 on the accumulation of hRAD51–ADP complexes, hRAD51-ssDNA filaments were incubated with or without mouse HOP2-MND1 (mHOP2-MND1) in the presence of Ca 2+ or Mg 2+ and [α- 32 P]ATP. The filaments were isolated on Nytran filters, and their nucleotide content was analysed by TLC [39] , [40] . The results showed no significant effect of mHOP2-MND1 on the accumulation of the hRAD51-ADP fraction in the presence of Ca 2+ or various Mg 2+ concentrations ( Fig. 1a–c ), even though mHOP2-MND1 has a small inhibitory effect on ATP hydrolysis by hRAD51 ( Supplementary Fig. 1 ). 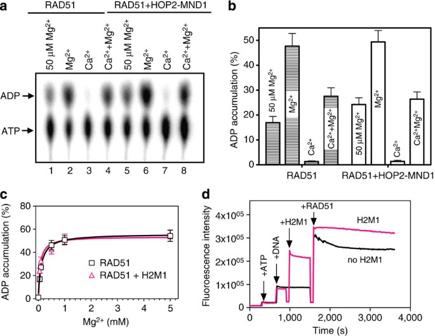Figure 1: HOP2-MND1 does not prevent the accumulation of RAD51-ADP complexes, but stabilizes the filament in an active form. (a) hRAD51 (10 μM) was added to ssDNA (#186, 30 μM) or to a mixture of ssDNA with mHOP2-MND1 (1 μM) in the presence of [α-32P]ATP and indicated metal ions. hRAD51 nucleoprotein complexes were isolated on Nytran filters and the ATP/ADP content was analysed by TLC39. (b) Graphical representation of data from (a). (c) Effect of Mg2+concentrations on hRAD51-ADP accumulation was measured as in (a). The concentrations of Mg2+and Ca2+were 1 mM, each, or 50 μM (when indicated). (d) The effect of mHOP2-MND1 on the fluorescence of hRAD51 complexes with etheno M13 ssDNA in the absence (denoted as ‘no H2M1’) or presence of mHOP2-MND1 (0.2 μM) (denoted as ‘H2M1’). The experiments were repeated at least three times; error bars indicate s.e.m. Figure 1: HOP2-MND1 does not prevent the accumulation of RAD51-ADP complexes, but stabilizes the filament in an active form. ( a ) hRAD51 (10 μM) was added to ssDNA (#186, 30 μM) or to a mixture of ssDNA with mHOP2-MND1 (1 μM) in the presence of [α- 32 P]ATP and indicated metal ions. hRAD51 nucleoprotein complexes were isolated on Nytran filters and the ATP/ADP content was analysed by TLC [39] . ( b ) Graphical representation of data from ( a ). ( c ) Effect of Mg 2+ concentrations on hRAD51-ADP accumulation was measured as in ( a ). The concentrations of Mg 2+ and Ca 2+ were 1 mM, each, or 50 μM (when indicated). ( d ) The effect of mHOP2-MND1 on the fluorescence of hRAD51 complexes with etheno M13 ssDNA in the absence (denoted as ‘no H2M1’) or presence of mHOP2-MND1 (0.2 μM) (denoted as ‘H2M1’). The experiments were repeated at least three times; error bars indicate s.e.m. Full size image It is known that formation of an active hRAD51-ssDNA filament in the presence of ATP causes stretching of ssDNA. Using etheno-ssDNA, a fluorescent derivative of ssDNA, this change in the ssDNA structure can be visualized by an increase in fluorescence. We previously showed that accumulation of ADP by the hRAD51-ssDNA in the presence of Mg 2+ causes a gradual decline in etheno-ssDNA fluorescence [39] . This decline, however, can be prevented by the inhibition of ATP hydrolysis in the presence of Ca 2+ . Here, we tested the effect of mHOP2-MND1 on the fluorescence of hRAD51 nucleoprotein complexes formed in the presence of mHOP2-MND1 and Mg 2+ . We found that mHOP2-MND1 prevented the decline in fluorescence almost completely, indicating preservation of the active hRAD51-ssDNA state. Thus, in contrast to Ca 2+ , mHOP2-MND1 does not suppress accumulation of ADP in the hRAD51 nucleoprotein filament. However, in spite of the accumulation of ADP mHOP2-MND1 was able to maintain the hRAD51-ssDNA filament in a ‘high-affinity’ active state proficient in DNA strand exchange. Still, the presence of triphosphate nucleosides was essential for mHOP2-MND1 stimulation of DNA strand exchange by hRAD51, as neither ADP nor AMP supported the reaction ( Supplementary Fig. 2 ). HOP2-MND1 stimulates RAD51 DNA strand exchange at low Mg 2+ We noticed that independently of mHOP2-MND1 the fraction of hRAD51–ADP complexes was decreased at low Mg 2+ (≤0.1 mM) and remained below 30% of total hRAD51–ATP/ADP complexes ( Fig. 1a (lanes 1 and 5) ), a level that is not inhibitory for DNA strand exchange [39] . This decrease in hRAD51–ADP complexes at low Mg 2+ concentration is consistent with a decrease in the hRAD51-binding affinity for ADP at low Mg 2+ (ref. 41 ). Here, we examined whether low Mg 2+ concentrations also stimulate DNA pairing by hRAD51. Using the D-loop assay that measures the ssDNA invasion into supercoiled dsDNA ( Fig. 2a ) we found that in the absence of mHOP2-MND1, Mg 2+ at low concentrations (0.05–0.5 mM) showed only slight stimulation of hRAD51 DNA strand exchange ( Fig. 2b,c ). Addition of mHOP2-MND1 caused strong stimulation of D-loop formation with the maximal yield observed at 0.025–0.1 mM Mg 2+ ( Fig. 2b,c ). As the experiments described above were performed with human RAD51 and mouse HOP2-MND1, we wanted to confirm our findings on mouse RAD51 (mRAD51), which differs from hRAD51 by four amino-acid substitutions. Indeed, using mRAD51 we observed the same dependence of simulation of D-loop formation by mHOP2-MND1 on Mg 2+ concentrations that was observed for hRAD51 ( Supplementary Fig. 3 ). Thus, mHOP2-MND1 in combination with low Mg 2+ concentrations showed the strongest stimulation of RAD51 DNA strand exchange. 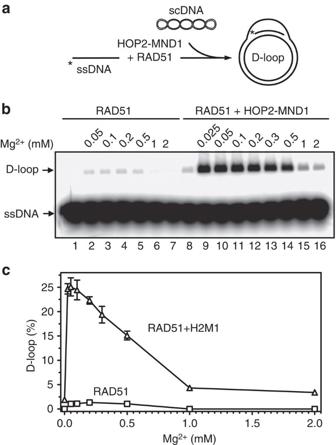Figure 2: HOP2-MND1 strongly stimulates D-loop formation at low Mg2+concentration. (a) The scheme of D-loop formation. The asterisk indicates32P label. (b) Effect of mHOP2-MND1 (0.1 μM) on D-loop formation by hRAD51 (1 μM) with pUC19 scDNA (50 μM) and ssDNA (#186, 3 μM) in buffer containing Mg2+at the indicated concentrations. D-loop formation was analysed by electrophoresis in a 1% agarose gel. Molecular size markers: D-loops (pUC19; 2,686 bp) and ssDNA (#186; 120 nt) are indicated by arrows. (c) Data from (b) are shown as a graph. The experiments were repeated at least three times; error bars indicate s.e.m. Figure 2: HOP2-MND1 strongly stimulates D-loop formation at low Mg 2+ concentration. ( a ) The scheme of D-loop formation. The asterisk indicates 32 P label. ( b ) Effect of mHOP2-MND1 (0.1 μM) on D-loop formation by hRAD51 (1 μM) with pUC19 scDNA (50 μM) and ssDNA (#186, 3 μM) in buffer containing Mg 2+ at the indicated concentrations. D-loop formation was analysed by electrophoresis in a 1% agarose gel. Molecular size markers: D-loops (pUC19; 2,686 bp) and ssDNA (#186; 120 nt) are indicated by arrows. ( c ) Data from ( b ) are shown as a graph. The experiments were repeated at least three times; error bars indicate s.e.m. Full size image HOP2-MND1 circumvents the requirement of RAD51 for Me 2+ During DNA strand exchange divalent metal ions (Me 2+ ) are needed mainly for complex formation with ATP molecules, which facilitates their binding to RAD51 (ref. 42 ). Therefore, we hypothesized that mHOP2-MND1 may substitute for Me 2+ , for example, by enhancing hRAD51 interactions with ATP. We tested this proposal by omitting Me 2+ from the reaction completely. To eliminate possible traces of Me 2+ , EDTA (0.5 mM) was added to the reactions. We found that indeed mHOP2-MND1 can induce D-loop formation by hRAD51 in the absence of Me 2+ ( Fig. 3a,b ). Importantly, the reaction required elevated ATP concentrations (>3 mM; with the maximum at 10 mM), indicating that ATP binding was the limited step during DNA strand exchange in the absence of Me 2+ . In contrast, hRAD51 alone did not promote DNA strand exchange in the absence of Me 2+ at any ATP concentration tested ( Fig. 3 ). Similarly, mHOP2-MND1 stimulated D-loop formation by mRAD51 in the absence of Me 2+ ( Supplementary Fig. 4 ). We conclude that mHOP2-MND1 can substitute for Me 2+ by promoting ATP binding to RAD51. 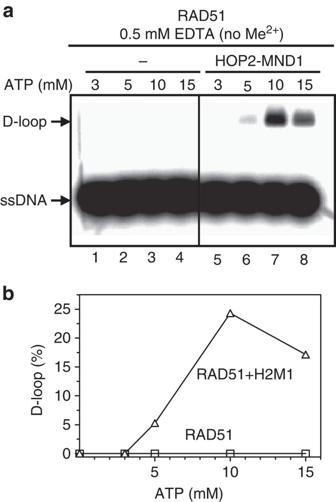Figure 3: HOP2-MND1 enables RAD51 DNA strand exchange in the absence of divalent metal ions. (a) Effect of mHOP2-MND1 (0.1 μM) on D-loop formation by hRAD51 (1 μM) with ssDNA (#186, 3 μM) and pUC19 scDNA (50 μM) in the presence of ATP at the indicated concentrations. D-loop formation was analysed by electrophoresis in a 1% agarose gel. (b) Data from (a) are shown as a graph. The experiments were repeated at least three times. Figure 3: HOP2-MND1 enables RAD51 DNA strand exchange in the absence of divalent metal ions. ( a ) Effect of mHOP2-MND1 (0.1 μM) on D-loop formation by hRAD51 (1 μM) with ssDNA (#186, 3 μM) and pUC19 scDNA (50 μM) in the presence of ATP at the indicated concentrations. D-loop formation was analysed by electrophoresis in a 1% agarose gel. ( b ) Data from ( a ) are shown as a graph. The experiments were repeated at least three times. Full size image HOP2-MND1 activates RAD51 K133A by enhancing its ATP binding The K133A mutation in hRAD51 strongly suppresses ATP binding, thereby inactivating DNA strand exchange in vitro [43] , [44] . As hRAD51 K133A is proficient in its interaction with mHOP2-MND1 (ref. 37 ) we tested whether mHOP2-MND1 can rescue the DNA strand exchange activity of hRAD51 K133A by stimulating its ATP binding. The DNA strand exchange activity of hRAD51 K133A was measured using the D-loop assay ( Fig. 2a ). While, as expected, no DNA strand exchange was observed in the absence of mHOP2-MND1 ( Fig. 4a , lanes 1–4), addition of mHOP2-MND1 activated DNA strand exchange activity of hRAD51 K133A ( Fig. 4a , lanes 5–8). The stimulatory effect was even stronger than for wild-type hRAD51, probably due to the fact that, in contrast to wild-type hRAD51, the hRAD51 K133A does not accumulate ADP within the filament. The reaction required elevated Mg 2+ concentrations (>0.5 mM). In contrast to wild-type hRAD51, DNA strand exchange promoted by hRAD51 K133A was not supported by Ca 2+ ( Fig. 4b ). 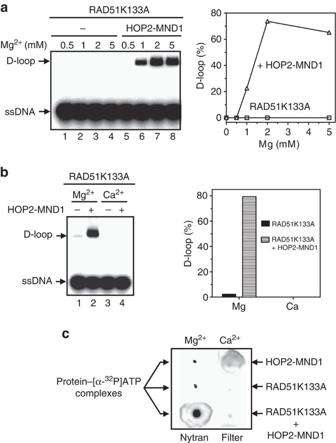Figure 4: HOP2-MND1 stimulates the DNA strand exchange activity of RAD51 K133A. (a) hRAD51 K133A (1 μM) was mixed with ssDNA (#90, 3 μM) in the absence (lanes 1–4) or in the presence of mHOP2-MND1 (0.1 μM) (lanes 5–8) and the indicated concentrations of Mg2+. The reactions were initiated by addition of pUC19 scDNA (50 μM). Analysis of D-loop formation by electrophoresis in a 1% agarose gel and the graphical representation of the data are shown on the left and right panels, respectively. (b) mHOP2-MND1 stimulates the DNA strand exchange activity of hRAD51K133A in the presence of Mg2+(2 mM), but not Ca2+(2 mM). (c) mHOP2-MND1 stimulates ATP binding by the hRAD51K133A-ssDNA filament in the presence of Mg2+. The efficiency of [α-32P]ATP binding by hRAD51 K133A was analysed by filter binding. mHOP2-MND1 (1 μM), hRAD51 K133A (10 μM) or mHOP2-MND1 and then hRAD51 K133A were incubated with ssDNA (#90, 30 μM) in the presence of [α-32P]ATP and Mg2+(2 mM) or Ca2+(2 mM) followed by filtration through a Nytran membrane. The experiments were repeated at least three times. Figure 4: HOP2-MND1 stimulates the DNA strand exchange activity of RAD51 K133A. ( a ) hRAD51 K133A (1 μM) was mixed with ssDNA (#90, 3 μM) in the absence (lanes 1–4) or in the presence of mHOP2-MND1 (0.1 μM) (lanes 5–8) and the indicated concentrations of Mg 2+ . The reactions were initiated by addition of pUC19 scDNA (50 μM). Analysis of D-loop formation by electrophoresis in a 1% agarose gel and the graphical representation of the data are shown on the left and right panels, respectively. ( b ) mHOP2-MND1 stimulates the DNA strand exchange activity of hRAD51K133A in the presence of Mg 2+ (2 mM), but not Ca 2+ (2 mM). ( c ) mHOP2-MND1 stimulates ATP binding by the hRAD51K133A-ssDNA filament in the presence of Mg 2+ . The efficiency of [α- 32 P]ATP binding by hRAD51 K133A was analysed by filter binding. mHOP2-MND1 (1 μM), hRAD51 K133A (10 μM) or mHOP2-MND1 and then hRAD51 K133A were incubated with ssDNA (#90, 30 μM) in the presence of [α- 32 P]ATP and Mg 2+ (2 mM) or Ca 2+ (2 mM) followed by filtration through a Nytran membrane. The experiments were repeated at least three times. Full size image We then assessed directly the effect of mHOP2-MND1 on ATP binding by hRAD51 K133A using filter binding ( Fig. 4c ) [39] , [40] . In accord with previous reports [43] , [44] , ATP binding by the hRAD51 K133A alone was inefficient, as almost no [α- 32 P]ATP–hRAD51 K133A complexes were retained on filters. In control experiments we showed that hRAD51K133A–ssDNA complexes were efficiently retained on the filters ( Supplementary Fig. 5 ). Addition of mHOP2-MND1 substantially stimulated ATP binding by hRAD51 K133A. Importantly, ATP binding and DNA strand exchange showed the same requirements for Me 2+ , it was supported by Mg 2+ , but not Ca 2+ ( Fig. 4b,c ). These results indicate that mHOP2-MND1 activates the DNA strand exchange activity of hRAD51 K133A by stimulating its interaction with ATP. The observed activation of hRAD51 K133A by mHOP2-MND1 may provide at least one possible rationalization to previous finding that hRAD51 K133A shows a degree of functionality in DSB repair in human cells in spite of the lack of DNA strand exchange activity in vitro [44] . HOP2-MND1 modifies the RAD51 preference for nucleotides During ATP hydrolysis, RAD51 binds ATP in the ground-state conformation. Then, upon nucleophilic attack by a water molecule ATP assumes the transition-state conformation. Here, we analysed which of these two conformations of hRAD51–ATP complex is susceptible for activation by mHOP2-MND1. We used two nucleotide cofactors, ADP-BeF 3 and ADP-AlF 4 , which in a vast majority of studied protein complexes mimicked the ground and transition states of ATP molecule, respectively [45] , [46] . In the absence of mHOP2-MND1 only ADP-AlF 4 , but not ADP-BeF 3 , supported DNA strand exchange under the conditions tested, indicating an important role of the ATP transition state for activation of the DNA strand exchange activity of hRAD51 ( Fig. 5a ; lanes 1 and 2). However, in the presence of mHOP2-MND1 both ADP-AlF 4 and ADP-BeF 3 efficiently supported DNA strand exchange ( Fig. 5a ; lanes 3 and 4). 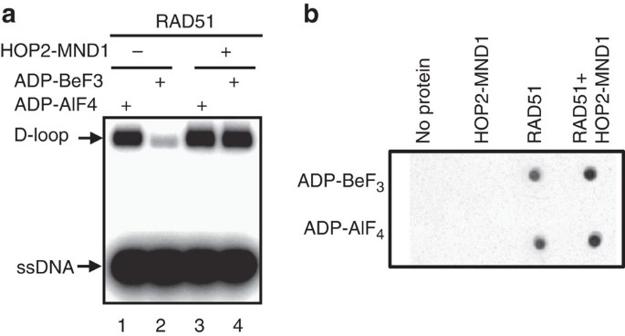Figure 5: HOP2-MND1 stimulates the DNA strand exchange activity of RAD51 in the presence of ADP-BeF3, a ground-state ATP analogue. (a) hRAD51 (1 μM) was incubated with ssDNA (#90, 3 μM) with or without mHOP2-MND1 (0.2 μM) in a reaction mixture containing either ADP-BeF3or ADP-AlF4. D-loop formation was initiated by addition of pUC19 scDNA. Molecular size markers: D-loops (pUC19; 2686, bp) and ssDNA (#90; 90 nt) are indicated by arrows. (b) Binding of [α-14C]ADP-AlF4and [α-14C]ADP-BeF3by hRAD51 (10 μM) in the absence or presence of mHOP2-MND1 (1 μM) was analysed by filter binding. mHOP2-MND1, hRAD51 or mHOP2-MND1 and then hRAD51 were incubated with ssDNA (#71, 30 μM) in the presence of Mg2+(0.1 mM) followed by filtration through Nytran membrane. The experiments were repeated at least three times. Figure 5: HOP2-MND1 stimulates the DNA strand exchange activity of RAD51 in the presence of ADP-BeF 3 , a ground-state ATP analogue. ( a ) hRAD51 (1 μM) was incubated with ssDNA (#90, 3 μM) with or without mHOP2-MND1 (0.2 μM) in a reaction mixture containing either ADP-BeF 3 or ADP-AlF 4 . D-loop formation was initiated by addition of pUC19 scDNA. Molecular size markers: D-loops (pUC19; 2686, bp) and ssDNA (#90; 90 nt) are indicated by arrows. ( b ) Binding of [α- 14 C]ADP-AlF 4 and [α- 14 C]ADP-BeF 3 by hRAD51 (10 μM) in the absence or presence of mHOP2-MND1 (1 μM) was analysed by filter binding. mHOP2-MND1, hRAD51 or mHOP2-MND1 and then hRAD51 were incubated with ssDNA (#71, 30 μM) in the presence of Mg 2+ (0.1 mM) followed by filtration through Nytran membrane. The experiments were repeated at least three times. Full size image We considered two non-exclusive hypotheses: mHOP2-MND1 may specifically enhance binding of ADP-BeF 3 to hRAD51 or it may force the hRAD51–ADP–BeF 3 complex into an active conformation for DNA strand exchange. Using the filter binding assay and 14 C-labelled ADP we found that ADP-AlF 4 and ADP-BeF 3 bind to hRAD51 with similar efficiency and that mHOP2-MND1 indeed stimulated nucleotide binding by hRAD51 ( Fig. 5b ). However, the stimulation was approximately the same (~2.0-fold) for ADP-AlF 4 and ADP-BeF 3 and therefore alone could not account for the specificity in DNA strand exchange stimulation by mHOP2-MND1 in the presence of ADP-BeF 3 . We conclude that mHOP2-MND1 both increases the affinity of hRAD51 for nucleotide cofactors and promotes conversion of the hRAD51-nucleoprotein filament to the active DNA strand exchange conformation. This conformational transition is apparently a key step in stimulation of hRAD51 DNA strand exchange activity by mHOP2-MND1. HOP2-MND1 increases RAD51 binding preference for ssDNA Unlike RecA, which preferentially binds ssDNA, RAD51 (human or yeast) shows similar affinities for ssDNA and dsDNA under normal conditions [47] . Therefore, auxiliary factors may be required to initiate DNA strand exchange in vivo , where both ssDNA and dsDNA are present. It has been shown that BRCA2 can specifically load hRAD51 on ssDNA [47] , [48] . We propose that mHOP2-MND1 by modulating hRAD51 interactions with nucleotide cofactors may also affect its DNA-binding specificity, because nucleotide cofactors are well-known regulators of hRAD51 DNA binding [39] , [49] . A direct link between nucleotide and DNA binding was previously demonstrated for RecA protein, the E. coli ortholog of hRAD51 (refs 50 , 51 ). Here, we investigated the effect of mHOP2-MND1 on the specificity of DNA binding by hRAD51 ( Fig. 6a ). 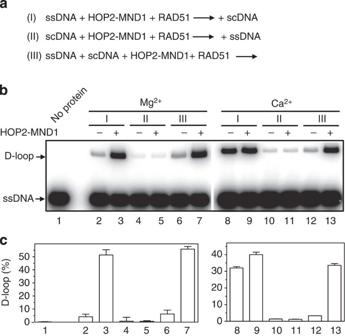Figure 6: The effect of the order of addition of DNA substrates on DNA strand exchange promoted by RAD51 in the presence or absence of HOP2-MND1. (a) Experimental scheme. (b) The nucleoprotein filaments were assembled by adding hRAD51 and mHOP2-MND1, when indicated, to ssDNA (I), scDNA (II) or mixture of ss- and scDNA (III) in the presence of Ca2+(0.85 mM) or Mg2+(0.5 mM). Reactions I and II were started by adding scDNA or ssDNA, respectively. D-loop formation was analysed by electrophoresis in 1% agarose gels. Molecular size markers: D-loops (pUC19; 2686, bp) and ssDNA (#90; 90 nt) are indicated by arrows. (c) Graphical representation of the data from (b). The experiments were repeated at least three times; the s.e.m. was within 10%. Figure 6: The effect of the order of addition of DNA substrates on DNA strand exchange promoted by RAD51 in the presence or absence of HOP2-MND1. ( a ) Experimental scheme. ( b ) The nucleoprotein filaments were assembled by adding hRAD51 and mHOP2-MND1, when indicated, to ssDNA (I), scDNA (II) or mixture of ss- and scDNA (III) in the presence of Ca 2+ (0.85 mM) or Mg 2+ (0.5 mM). Reactions I and II were started by adding scDNA or ssDNA, respectively. D-loop formation was analysed by electrophoresis in 1% agarose gels. Molecular size markers: D-loops (pUC19; 2686, bp) and ssDNA (#90; 90 nt) are indicated by arrows. ( c ) Graphical representation of the data from ( b ). The experiments were repeated at least three times; the s.e.m. was within 10%. Full size image We found that mHOP2-MND1 stimulates DNA strand exchange when hRAD51 was added to the mixture of ssDNA (3 μM) and pUC19 supercoiled dsDNA (scDNA) (50 μM) substrates (reaction III) in the presence of either Mg 2+ or Ca 2+ ( Fig. 6b,c ; lanes 7 and 13). The efficiency of this reaction was similar to the ‘conventional’ one that was initiated by pre-incubating hRAD51 with ssDNA (reaction I) ( Fig. 6b,c ; lanes 3 and 9). In contrast, pre-incubation of both hRAD51 and mHOP2-MND1 with pUC19 scDNA (reaction II) did not yield D-loops, indicating that mHOP2-MND1 and hRAD51 in the absence of ssDNA may form stable complexes with dsDNA that are non-productive in DNA strand exchange ( Fig. 6b,c ; lanes 5 and 11). The experiments with mRAD51 yielded similar results ( Supplementary Fig. 6 ). Taken together, our current data show that mHOP2-MND1 may specifically help RAD51 to form filament on ssDNA even in the presence of a large excess of dsDNA. HOP2-MND1 prevents RAD51 inhibition by non-homologous ssDNA It was previously shown that non-homologous ssDNA inhibits DNA strand exchange promoted by RecA by competing with dsDNA for the RecA secondary binding site during the search for homology [16] , [17] . Here, we examined whether ssDNA causes a similar inhibition of the DNA strand exchange promoted by hRAD51 and how mHOP2-MND1 would affect this inhibition ( Fig. 7a ). 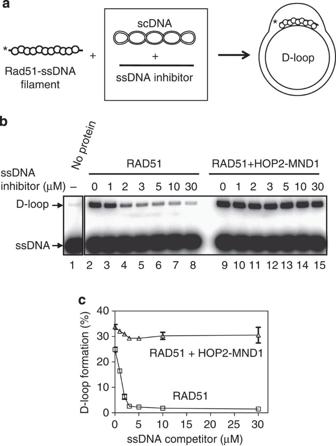Figure 7: HOP2-MND1 alleviates RAD51 inhibition by non-homologous ssDNA. (a) The scheme of the reaction. The asterisk indicates32P label on the ssDNA. (b) Analysis of the D-loops in agarose gels. The nucleoprotein filaments were formed by incubating hRAD51 (1 μM) with32P-ssDNA (#90, 3 μM) in standard buffer containing 1 mM ATP and 0.85 mM Ca2+with or without mHOP2-MND1 (200 nM). The reactions were initiated by addition of pUC19 scDNA premixed with a non-homologous ssDNA inhibitor (#71) (at the indicated concentrations). Molecular size markers: D-loops (pUC19; 2,686 bp) and ssDNA (#90; 90 nt) are indicated by arrows. (c) Data from (b) shown as a graph. The experiments were repeated at least three times; error bars indicate s.e.m. Figure 7: HOP2-MND1 alleviates RAD51 inhibition by non-homologous ssDNA. ( a ) The scheme of the reaction. The asterisk indicates 32 P label on the ssDNA. ( b ) Analysis of the D-loops in agarose gels. The nucleoprotein filaments were formed by incubating hRAD51 (1 μM) with 32 P-ssDNA (#90, 3 μM) in standard buffer containing 1 mM ATP and 0.85 mM Ca 2+ with or without mHOP2-MND1 (200 nM). The reactions were initiated by addition of pUC19 scDNA premixed with a non-homologous ssDNA inhibitor (#71) (at the indicated concentrations). Molecular size markers: D-loops (pUC19; 2,686 bp) and ssDNA (#90; 90 nt) are indicated by arrows. ( c ) Data from ( b ) shown as a graph. The experiments were repeated at least three times; error bars indicate s.e.m. Full size image The results show that addition of non-homologous ssDNA together with pUC19 scDNA to the hRAD51-ssDNA filament strongly inhibits D-loop formation ( Fig. 7b (lanes 2 ). This inhibition was rescued by RPA, when it was added after ssDNA, indicating that inhibition was indeed caused by binding of ssDNA to the secondary hRAD51 site and not by relocation of hRAD51 to ssDNA-inhibitor ( Supplementary Fig. 7 ). We tested then the effect of mHOP2-MND1 on the inhibition of DNA strand exchange caused by ssDNA. The inhibition was completely abolished in the presence of mHOP2-MND1 ( Fig. 7b (lanes 10 ) regardless of whether mHOP2-MND1 was added to hRAD51 filament before or after non-homologous ssDNA ( Supplementary Fig. 8 ; lanes 3 and 5). It is unlikely that mHOP2-MND1 exerts its effect by capturing an excess of ssDNA-inhibitor because the amount of ssDNA significantly exceeded the mHOP2-MND1-binding capacity (see Discussion). In contrast, addition of homologous (complementary) ssDNA to the hRAD51-ssDNA filament inhibited DNA strand exchange even in the presence of mHOP2-MND1 most likely due to its annealing with ssDNA residing within the hRAD51 primary site and formation of dsDNA that is inactive in DNA strand exchange with pUC19 scDNA ( Supplementary Fig. 8 ; lanes 2, 4 and 6). This result is consistent with the known ssDNA-annealing activity of hRAD51 and mHOP2-MND1 (refs 34 , 52 ) and indicates that mHOP2-MND1 does not impair accessibility of the hRAD51-ssDNA filament for ssDNA. Thus, the current results demonstrate a strong effect of mHOP2-MND1 on the DNA-binding specificity of the hRAD51-ssDNA filament. mHOP2-MND1 specifically promotes binding of the hRAD51 to dsDNA during the homology search by rendering it resistant to inhibition with non-homologous ssDNA. HOP2-MND1 affects the conformation of RAD51 To rationalize the effects of mHOP2-MND1 on various RAD51 activities observed in our study we suggested that mHOP2-MND1 by acting through physical interaction [33] , [34] , [36] may trigger a shift in RAD51 folding towards a conformation that favors formation of an active nucleoprotein filament. We tested the effect of mHOP2-MND1 on the hRAD51 conformation by analysing the pattern of hRAD51 digestion by proteases in the presence and absence of mHOP2-MND1. It is known that even small changes in protein folding can cause a significant change in this pattern [53] . Here, we analysed changes in the pattern of the hRAD51 fragments produced by trypsin in the presence of mHOP2-MND1, ssDNA and ATP by western blotting using antibodies specific for the His-tag at the N terminus of hRAD51. We found that hRAD51 alone is very sensitive to trypsin ( Fig. 8a ; lane 2). However, ssDNA had a protective effect on hRAD51 digestion, as evidenced by the fact that 13.5 times more of the full-length protein remained after digestion ( Fig. 8 ; lane 3). The protective effect of ssDNA was especially strong (22.5-fold protection) when it was combined with ATP, conditions that support formation of the hRAD51-ssDNA filament. The mHOP2–MND1 heterodimer also protected hRAD51 from tryptic digestion in the absence of DNA when added alone (threefold protection) or in the presence of ATP (twofold). 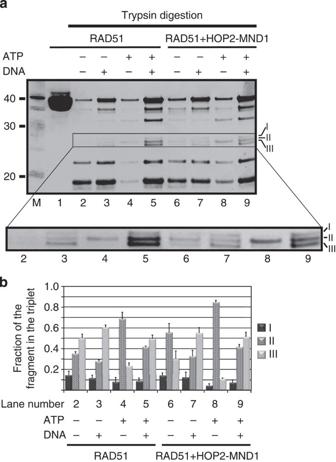Figure 8: HOP2-MND1 induces conformational changes upon interaction with RAD51. (a) His-hRAD51 (5 μM) was digested by trypsin (19 μg ml−1) in the absence (lanes 2–5) or presence of mHOP2-MND1 (0.5 μM; lanes 6–9). Where indicated the reaction contained ϕX174 ssDNA (15 μM, nucleotides) (lanes 3, 5, 7 and 9) and/or ATP (1 mM) (lanes 4, 5, 8 and 9). The hRAD51 fragments were resolved in a 12% NuPAGE Bis-Tris gel (Life Technologies) in MES buffer and visualized by western blotting using anti-HIS tag monoclonal antibody (Abgent). Numbers on the left indicate approximate size of the fragments (kDa) as determined by positions of His-tagged BenchMark markers. The region of the gel corresponding to a particular part of hRAD51 undergoing conformational changes upon addition of DNA or/and nucleotide cofactors is highlighted as enhanced in the inset. The fragments relevant to the discussion in the text are marked by roman numbers I, II and III. Untreated hRAD51 (38 kDa) is shown in lane 1. His-tagged BenchMark markers (Invitrogen) are denoted by ‘M’. (b) The relative intensity of each fragment shown in the inset is plotted as a fraction of the sum of intensities of fragments I–III. The digestion patterns were reproduced in four (for the trypsin digestion in the absence of mHOP2-MND1) or three (digestion in the presence of the HOP2–MND1 complex) independent experiments. Error bars represent the s.d. Figure 8: HOP2-MND1 induces conformational changes upon interaction with RAD51. ( a ) His-hRAD51 (5 μM) was digested by trypsin (19 μg ml −1 ) in the absence (lanes 2–5) or presence of mHOP2-MND1 (0.5 μM; lanes 6–9). Where indicated the reaction contained ϕX174 ssDNA (15 μM, nucleotides) (lanes 3, 5, 7 and 9) and/or ATP (1 mM) (lanes 4, 5, 8 and 9). The hRAD51 fragments were resolved in a 12% NuPAGE Bis-Tris gel (Life Technologies) in MES buffer and visualized by western blotting using anti-HIS tag monoclonal antibody (Abgent). Numbers on the left indicate approximate size of the fragments (kDa) as determined by positions of His-tagged BenchMark markers. The region of the gel corresponding to a particular part of hRAD51 undergoing conformational changes upon addition of DNA or/and nucleotide cofactors is highlighted as enhanced in the inset. The fragments relevant to the discussion in the text are marked by roman numbers I, II and III. Untreated hRAD51 (38 kDa) is shown in lane 1. His-tagged BenchMark markers (Invitrogen) are denoted by ‘M’. ( b ) The relative intensity of each fragment shown in the inset is plotted as a fraction of the sum of intensities of fragments I–III. The digestion patterns were reproduced in four (for the trypsin digestion in the absence of mHOP2-MND1) or three (digestion in the presence of the HOP2–MND1 complex) independent experiments. Error bars represent the s.d. Full size image Furthermore, we identified which hRAD51 tryptic fragments showed especially strong dependence on RAD51-interacting cofactors/partners ( Fig. 8a , inset). In the absence of either ATP or ssDNA, very little N-terminal hRAD51 fragments were generated in this region by trypsin ( Fig. 8a ; inset, lane 2). Addition of ssDNA led to the proportional enhancement of the intensities of fragments I–III with fragment III being the most intense ( Fig. 8a (inset, lane 3) ). Treatment of hRAD51 in the presence of ATP produced predominantly fragment II (68%, relative to the sum of intensities of I, II and III fragments) ( Fig. 8a (inset, lane 4) ), whereas treatment in the presence of both ssDNA and ATP (hRAD51–ssDNA–ATP complex) strongly enhanced fragments II and III (41 and 52%, respectively). Addition of mHOP2-MND1 to hRAD51 in the absence of ssDNA and ATP led to a very distinct tryptic pattern with fragment II being the most prominent (over 50%) that resembled the pattern of hRAD51 digestion produced without mHOP2-MND1 in the presence of ATP ( Fig. 8b , quantification of lanes 4 and 6). Intriguingly, digestion of hRAD51 in the presence of both ATP and mHOP2-MND1 increased the relative yield of fragment II even further (84%) ( Fig. 8a (lane 8) ). Thus, mHOP2-MND1 has a significant effect on the pattern of tryptic digestion of hRAD51 that may reflect conformational changes generated in hRAD51 by mHOP2-MND1. Moreover, the changes in the hRAD51 proteolysis pattern induced by mHOP2-MND1 paralleled those induced by ATP, suggesting similarities in the conformational alterations induced in hRAD51 by the nucleotide cofactor and the accessory protein. HOP2-MND1 plays an important role in HR by stimulating the DNA strand exchange activity of RAD51 and DMC1 (refs 33 , 36 , 37 ). We show that mHOP-MND1 has a profound and unique effect on properties of RAD51, modulating both the strength and the specificities of its interactions with nucleotide cofactors and DNA. Whereas our results demonstrate differences in the mechanisms of hRAD51 stimulation by mHOP2-MND1 and by Ca 2+ , there is a common component of these mechanisms: both Ca 2+ and mHOP2-MND1 target one of the most basic attributes of RAD51—its interactions with nucleotide cofactors. Thus, Ca 2+ prevents accumulation of ADP, maintaining the hRAD51 nucleoprotein in an ATP-bound active high-affinity state by inhibiting hRAD51 ATPase activity [39] . In contrast, mHOP2-MND1 does not affect the level of ADP, but nonetheless is able to maintain the hRAD51 filament in the same active high-affinity state. mHOP2-MND1 significantly enhances the binding affinity and broadens the specificity of hRAD51 interactions with nucleotide cofactors. Remarkably, mHOP2-MND1 enables hRAD51 or mRAD51 to bind ATP and promote DNA strand exchange in the absence of divalent metal ions, or is capable of inducing ATP binding and hence the DNA strand exchange activity of the hRAD51 K133A mutant that is deficient in ATP binding. In the presence of mHOP2-MND1, hRAD51 can efficiently utilize ADP˙BeF 3 , a ground-state ATP analogue, which poorly supports DNA strand exchange in the absence of HOP2-MND1 ( Fig. 5 ). These data indicate that mHOP2-MND1 imposes conformational changes forcing the hRAD51–ADP˙BeF 3 complex into an active conformation, similar to that of the complex with the transition-state analogue ADP˙AlF 4 . Such stabilization of the hRAD51–nucleotide complexes by mHOP2-MND1 in the transition-state conformation is consistent with a small inhibitory effect of mHOP2-MND1 on ATP hydrolysis by hRAD51 ( Supplementary Fig. 1 ). The dramatic change that mHOP2-MND1 brings about on the DNA binding specificity of RAD51 is remarkable. We have previously reported that mHOP2-MND1 promotes preferential binding of DMC1 to ssDNA from the mixture with dsDNA during nucleoprotein filament formation [33] . The current data show a similar mHOP2-MND1 effect on RAD51, underscoring similarities in the mechanisms of the stimulation of both recombinases by mHOP2-MND1. mHOP2-MND1 could affect RAD51-binding specificity by either promoting dissociation of RAD51–dsDNA complexes or enhancing RAD51 loading on ssDNA, for example, similar to BRCA2 (refs 47 , 48 , 54 ). The results of our order of addition experiments demonstrating the inability of mHOP2-MND1 to stimulate DNA strand exchange when RAD51 was pre-bound to dsDNA argue against the former mechanism. However, a simple mechanism of RAD51 loading on ssDNA by mHOP2-MND1 is not supported by the DNA-binding specificity of HOP2-MND1 that binds both ssDNA and dsDNA and shows a higher affinity for dsDNA [34] , [36] , [37] . We suggest that mHOP2-MND1 modulates changes in DNA-binding properties of RAD51 by modifying its conformation through physical interaction with this protein. Previously, it was reported that monovalent salts enhance RAD51/RecA-specific binding to ssDNA by inducing conformational changes in the protein [49] , [50] , [51] , [55] . We suggested that mHOP2-MND1 may also act by inducing conformational changes in RAD51 that foster the binding preferences of its primary and secondary sites for ssDNA and dsDNA, respectively. Indeed, our results with trypsin footprinting support this hypothesis demonstrating significant conformational changes induced in hRAD51 by mHOP2-MND1. In addition, some changes in the RAD51 proteolytic pattern induced by mHOP2-MND1 resembled those induced by ATP binding. We suggest that the conformational changes induced by mHOP2-MND1 are also responsible for the modulation of nucleotide binding by RAD51 observed in our experiments. Interestingly, a relatively low stoichiometric ratio of 1 mHOP2-MND1 heterodimer per 10 RAD51 monomers appeared to be sufficient for both the stimulation of DNA strand exchange and the induction of detectable conformational changes in RAD51. Thus, mHOP2-MND1 is capable of maintaining the RAD51-ssDNA filament in an active form by targeting a relatively small fraction of RAD51 monomers. We found that mHOP2-MND1 has another and unique effect on the DNA-binding specificity of RAD51; it renders the hRAD51-ssDNA filament insensitive to inhibition by non-homologous ssDNA. Previously, it was shown that the E. coli RecA, the best-studied member of the RecA/RAD51/RadA family, forms a nucleoprotein filament by binding ssDNA in the primary site and leaving its secondary site vacant for interaction with dsDNA during the search for homology. The secondary site, however, can bind both dsDNA and ssDNA, and shows a greater affinity for ssDNA [16] , [17] . It was suggested that the high affinity of the secondary site for ssDNA is instrumental for the search for homology, as it binds the ssDNA strand displaced from initial joint molecules causing their stabilization. However, because of a high ssDNA binding affinity of the secondary site, exogenous ssDNA can inhibit the search for homology by RecA by competing with dsDNA binding. Our current data demonstrate that the RAD51-promoted DNA strand exchange is also sensitive to ssDNA inhibition consistent with the evolutionary conservation of its mechanism. mHOP2-MND1 completely averts inhibition of DNA strand exchange by ssDNA that was at a 10-fold excess over the RAD51-ssDNA filament. It is unlikely that mHOP2-MND1 exerts its effect by capturing an excess of ssDNA-inhibitor in a manner similar to that of RPA. Previously, it was shown that mHOP2-MND1 binds ssDNA with an apparent stoichiometry of 1.2 nucleotides per heterodimer [34] . Thus, under our conditions, mHOP2-MND1 could capture only 0.8% of ssDNA-inhibitor present in the reaction mixture. HOP2-MND1 aversion of the inhibition of DNA strand exchange by ssDNA may have important biological implications. In both yeast and mice HOP2-MND1 mutations not only impair HR in meiosis but also show formation of synaptonemal complex between non-homologous chromosomes [25] , [26] , [32] . During meiosis, an excessive number of DSBs are formed and processed into ssDNA tails; 3–15 and 15–20 DSBs per homologous chromosome pair are estimated to form in yeast and mammals, respectively [56] . In the absence of HOP2-MND1, the search for homology and pairing of these ssDNA tails with homologous chromosomes is disrupted. However, they may still form complexes with the secondary site of the RAD51/DMC1 filaments on non-homologous chromosomes promoting non-homologous synapsis. While RPA/Ssb can disrupt these interactions, experiments with RecA showed that binding of ssDNA to the secondary site of the nucleoprotein filament is a very fast process [16] , and may occur before RPA/Ssb binding to ssDNA. Furthermore, in the context of the synaptonemal complex the joints between ssDNA and the secondary site may become inaccessible for RPA binding. Thus, HOP2-MND1 may facilitate synapsis of homologous chromosomes by two mechanisms: by stimulating RAD51/DMC1 strand exchange activity and by preventing deleterious non-homologous interactions between ssDNA and the RAD51/DMC1 filament. We propose that more experiments with Hop2 −/− and Mnd1 −/− cells are needed to establish the biological relevance of our current in vitro observations on the effect of RAD51 nucleotide and DNA binding caused by mHOP2-MND1. Proteins and DNA hRAD51, hRAD51 K133A and mRAD51 proteins were expressed as N-terminal His-tagged fusions in BLR21 ΔrecA E. coli cells (Novagene) using pET15b vector. Proteins were purified by ammonium sulphate precipitation (0.23 g of ammonium sulphate per 1 ml of cleared lysate) followed by chromatography on Ni-agarose, heparin Sepharose and MonoQ columns [39] . The mHOP2-MND1 was purified by coexpressing His-tagged mHOP2 protein and untagged mMND1 protein in Codon Plus PR strain (Stratagene) using pET15b vector followed by consecutive chromatographic steps on Ni-agarose, MonoQ, macro hydroxyapatite, heparin Sepharose and MonoS columns [33] . Supercoiled pUC19 dsDNA was prepared using plasmid purification kits (Qiagen). Oligonucleotides (IDT, Inc.) used in this study ( Supplementary Table 1 ) were purified by gel electrophoresis in polyacrylamide gels containing 50% urea, labelled with 32 P using T4 polynucleotide kinase (NEB) and [γ- 32 P]ATP, annealed and stored at −20 °C (ref 57 ). D-loop formation by RAD51 in the presence of HOP2-MND1 Reactions were carried out in standard buffer containing 25 mM Tris acetate (pH 7.5), 1 mM ATP (or indicated otherwise), CaCl 2 or magnesium acetate (at the indicated concentrations), 2 mM DTT, BSA (100 μg ml −1 ) and 32 P-labelled ssDNA (#90; 3 μM, nucleotides). First, 32 P-labelled ssDNA was incubated with mHOP2-MND1 heterodimer (100 nM, or indicated otherwise) for 5 min at 37 °C. Then, to form the nucleoprotein filament, human or mouse RAD51 protein (1 μM) was added and incubation continued for 15 min. Formation of D-loops was initiated by addition of pUC19 scDNA (50 μM, nucleotides). D-loop formation was terminated after a 15-min incubation. The DNA products were deproteinized by the addition of 1.5% SDS and proteinase K (1.6 mg ml −1 ) for 15 min at 37 °C, mixed with a 0.10 volume of loading buffer (70% glycerol, 0.1% bromphenol blue) and analysed by electrophoresis in 1% agarose gels in TAE buffer (40 mM Tris acetate (pH 8.3) and 1 mM EDTA) at 5 V cm −1 for 1.5 h. The gels were dried on DEAE-81 paper (Whatman) and quantified using a Storm 840 PhosphorImager and ImageQuant 5.2 (GE Healthcare). When indicated, alternative orders of addition of the reaction mixture components were used. Reactions in the absence of Me 2+ were supplemented with 0.5 mM EDTA. The reactions with hRAD51 K133A mutant were carried out in the presence of 2 mM magnesium acetate or 2 mM CaCl 2 , unless otherwise indicated. D-loop formation in the presence of ATP analogues The reactions were carried out in buffer containing 25 mM Tris acetate (pH 7.5) 2 mM ADP, 0.1 mM magnesium acetate, 25 mM NaCl and 25 mM KCl (from protein stocks), 2 mM DTT, BSA (100 μg ml −1 ), 32 P-labelled ssDNA (#90; 3 μM, nucleotides), 0.7 mM Al(NO 3 ) 3 or BeSO 4 , and 8 mM NaF. mHOP2-MND1 (100 nM) was incubated first with 32 P-labelled ssDNA for 5 min at 37 °C. hRAD51 (1 μM) was added then to the reaction mixture and incubation continued for 15 min. Formation of D-loops was initiated by addition of pUC19 scDNA (50 μM, nucleotides) and continued for 15 min. The DNA products were deproteinized, analysed by electrophoresis in a 1% agarose gel and visualized as described above. Fluorimetric assay Etheno M13 ssDNA (3 μM) was incubated in the absence or presence of mHOP2-MND1 (0.2 μM) in the buffer containing 33 mM Hepes (pH 7.0), 1 mM ATP, 1 mM DTT and 0.5 mM magnesium acetate for 10 min at 37 °C. Then, hRAD51 (1 μM) was added to the reaction mixture to initiate nucleoprotein filament formation. Fluorescence of etheno M13 ssDNA was excited at 300 nm and monitored at 408 nm using a FluoroMax-3 fluorometer (Jobin Yvon Inc). Measurement of ATP binding by RAD51 K133A The reaction mixtures contained 25 mM Tris acetate (pH 7.5), 0.2 mM ATP, 5 μCi [α- 32 P]ATP, 2 mM CaCl 2 or magnesium acetate, 2 mM DTT, BSA (100 μg ml −1 ) and ssDNA (#90; 30 μM, nucleotides). First, mHOP2-MND1 (1.3 μM) was incubated with ssDNA for 5 min at 37 °C. Then, hRAD51 K133A (10 μM) was added and incubation continued for 15 min. The resulting nucleoprotein complexes were subjected to vacuum filtration through Nylon membrane (Schleicher and Schuell). To remove unbound [α- 32 P]ATP, the membrane was washed with buffer containing 25 mM Tris acetate (pH 7.5) and either 2 mM CaCl 2 or 2 mM magnesium acetate. The membrane was dried and the amount of hRAD51-bound ATP was visualized and quantified using a Storm 840 PhosphorImager and ImageQuant 5.2 software (GE Healthcare). Measurement of ADP-AlF 4 and ADP-BeF 3 binding by RAD51 The reaction mixtures contained 25 mM Tris acetate (pH 7.5), 0.2 mM ADP, 5 μCi [ 14 C]ADP, 0.1 mM magnesium acetate, 2 mM DTT, BSA (100 μg ml −1 ), ssDNA (#90; 30 μM, nucleotides), 0.7 mM Al(NO 3 ) 3 or BeSO 4 , and 8 mM NaF. First, mHOP2-MND1 (1 μM) was incubated with ssDNA for 5 min at 37 °C. Then, hRAD51 (10 μM) was added and incubation continued for 15 min. The resulting nucleoprotein complexes were subjected to vacuum filtration through Nylon membrane (Schleicher and Schuell). To remove unbound [ 14 C]ADP, the membrane was washed twice with buffer containing 25 mM Tris acetate (pH 7.5) and 0.1 mM magnesium acetate. The membrane was dried and the amount of hRAD51-bound ATP was visualized and quantified using a Storm 840 PhosphorImager and ImageQuant 5.2 software (GE Healthcare). Treatment of RAD51 complexes with trypsin Reactions (20 μl) containing 25 mM Tris acetate (pH 7.5), 15 mM NaCl, 1 mM magnesium acetate, 2 mM DTT and 5 μM hRAD51 with the N-terminal His-tag were supplemented where indicated with 1 mM ATP, ϕX174 ssDNA (15 μM, nucleotides) and 0.5 μM mHOP2-MND1. The mHOP2–MND1 complex was purified as a His-tag fusion; the His-tag was removed by treatment with the Thrombin Cleavage Kit (Sigma-Aldrich) followed by additional purification on Ni-NTA (Qiagene) and MonoQ (GE Healthcare) columns. First, ssDNA was incubated with mHOP2-MND1 for 5 min at 37 °C and then with hRAD51 for additional 15 min. One microlitre of 400 μg ml −1 MS-Grade Pierce Trypsin Protease (Thermo Scientific) in 50 mM acetic acid was added to the reactions (final concentration of trypsin 19 μg ml −1 ) and the digestion proceeded for 40 min at 37 °C. Trypsin was inactivated by addition of 1 × NuPAGE LDS Sample Buffer (Life Technologies) with 20 mM DTT and heating for 10 min at 70 °C. The samples along with His-tagged BenchMark markers (Invitrogen) were separated in a 12% NuPAGE Bis-Tris gel (Life Technologies) in MES buffer. Protein fragments were transferred to a PVDF membrane (Life Technologies) with Trans-Blot Semi-Dry electrophoretic transfer cell (Bio-Rad). The N-terminal fragments of hRAD51 containing His-tags were detected using purified mouse anti-HIS tag monoclonal antibody (Abgent) and Alexa Fluor 680 goat anti-mouse IgG. The fluorescent intensities were measured with a FLA-9000 image scanner (FujiFilm) using the Science Lab Multi Gauge 3.2 Software (FujiFilm). The region of the gel containing three hRAD51 fragments (I–III), the generation of which showed a high sensitivity to hRAD51 conformational changes upon addition of DNA or/and nucleotide cofactors, was identified ( Fig. 8 ). After quantification, the relative fluorescence intensity of each of these fragments was calculated and plotted as a fraction of the sum of the fluorescence intensities of fragments I–III for each experimental condition ( Fig. 8b ). How to cite this article: Bugreev, D. V. et al. HOP2-MND1 modulates RAD51 binding to nucleotides and DNA. Nat. Commun. 5:4198 doi: 10.1038/ncomms5198 (2014).